N2activation on a molybdenum–titanium–sulfur cluster The FeMo-cofactor of nitrogenase, a metal–sulfur cluster that contains eight transition metals, promotes the conversion of dinitrogen into ammonia when stored in the protein. Although various metal–sulfur clusters have been synthesized over the past decades, their use in the activation of N 2 has remained challenging, and even the FeMo-cofactor extracted from nitrogenase is not able to reduce N 2 . Herein, we report the activation of N 2 by a metal–sulfur cluster that contains molybdenum and titanium. An N 2 moiety bridging two [Mo 3 S 4 Ti] cubes is converted into NH 3 and N 2 H 4 upon treatment with Brønsted acids in the presence of a reducing agent. Metal–sulfur clusters are a ubiquitous class of inorganic compounds, and span a wide range of structural and electronic features [1] , [2] . One unique function of protein-supported clusters is the conversion of N 2 into NH 3 , which is mediated by the FeMo-cofactor of nitrogenase (Fig. 1 a) [3] , [4] , [5] . The FeMo-cofactor can be extracted from the protein into organic solvents without significant degradation of its metal–sulfur core [6] , [7] . The extracted form catalyzes the reduction of non-native C 1 substrates, such as CO and CO 2 in the presence of reducing agents and protons to furnish CH 4 and short-chain hydrocarbons [8] , [9] , and similar catalytic reductions can also be accomplished with the synthetic analog [Cp*MoFe 5 S 9 (SH)] 3– (Cp* = η 5 -C 5 Me 5 ) [10] . However, N 2 cannot be reduced with the extracted FeMo-cofactor [7] or its synthetic analogs, highlighting the difference in N 2 -reducing activity between the protein-supported FeMo-cofactor and discrete metal–sulfur clusters in solution. Thus, a molecular basis for the reduction of N 2 on metal–sulfur clusters remains elusive, while some aqueous suspensions or emulsions of Fe–S or Mo–Fe–S compounds have been found to generate NH 3 [11] , [12] , [13] , [14] and some thiolate-supported Fe complexes have been found to activate N 2 [15] , [16] , [17] . The cuboidal cluster Cp* 3 Ir 3 S 4 Ru(tmeda)(N 2 ) (tmeda = tetramethylethylenediamine) is the only structurally characterized example for the binding of N 2 to a metal–sulfur cluster, although the conversion of the Ru-bound N 2 has not yet been achieved [18] . Fig. 1 Structure of the nitrogenase FeMo-cofactor. a The resting-state structure. The peptide chains of cysteine (Cys) and histidine (His), as well as a part of ( R )-homocitrate are omitted for clarity. Color legend: C, gray; Fe, black; Mo, dark blue; S, yellow; O, red; N, light blue. b Wire-frame drawing of the inorganic part of the FeMo-cofactor, which highlights the fused form of the two cubes Full size image It should be noted that the structure of the FeMo-cofactor can be seen as a fused form of two cubes (Fig. 1b ), implying the utility of cubes in the activation of N 2 . However, synthetic examples are limited for the fused form of such metal–sulfur cubes [19] , [20] , [21] , [22] , [23] , and a carbon-centered derivative still remains unprecedented. In order to develop a strategy for the activation of N 2 on synthetic metal–sulfur clusters, we examined independent cubes in this study. Our design (Fig. 2 ) is based on the trinuclear Mo–sulfur cluster platform Cp* 3 Mo 3 (μ-S) 3 (μ 3 -S) ( 1 ) [24] for the accommodation of a metal atom via three doubly bridging sulfur atoms to furnish a cubic structure. Ti was chosen as the additional metal to demonstrate the proof-of-concept, on the basis of successful examples of Ti complexes in N 2 chemistry [25] , e.g. some recent studies on the activation of N 2 mediated by Ti–hydride complexes [26] , [27] . The resulting [Mo 3 S 4 Ti] cluster (Fig. 2 , top right) is reduced in the presence of N 2 , to generate a Ti-based reaction site for the activation of N 2 . Herein, we report the activation of N 2 , as well as its conversion into NH 3 and N 2 H 4 , on a Mo–Ti–S cluster. Fig. 2 Reactions in this study. Synthesis of the cubic [Mo 3 S 4 Ti] cluster 2 , the N 2 -binding cluster 3 , and its 1e reduced form [ 3 ] – ; Cp* = η 5 -pentamethylcyclopentadienyl; THF tetrahydrofuran Full size image Synthesis of a cubic [Mo 3 S 4 Ti] cluster and an N 2 -cluster The cubic [Mo 3 S 4 Ti] precursor cluster Cp* 3 Mo 3 S 4 TiCl 2 ( 2 ) was synthesized in 70% yield in tetrahydrofuran (THF) from the reaction of in situ generated [ 1 ] – with TiCl 3 (THF) 3 (Fig. 2 ), in a manner similar to the synthesis of cubic clusters from trinuclear Mo–sulfur clusters [28] , [29] . 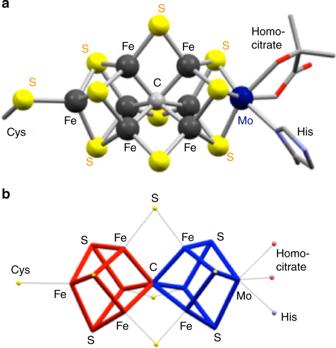Fig. 1 Structure of the nitrogenase FeMo-cofactor.aThe resting-state structure. The peptide chains of cysteine (Cys) and histidine (His), as well as a part of (R)-homocitrate are omitted for clarity. Color legend: C, gray; Fe, black; Mo, dark blue; S, yellow; O, red; N, light blue.bWire-frame drawing of the inorganic part of the FeMo-cofactor, which highlights the fused form of the two cubes 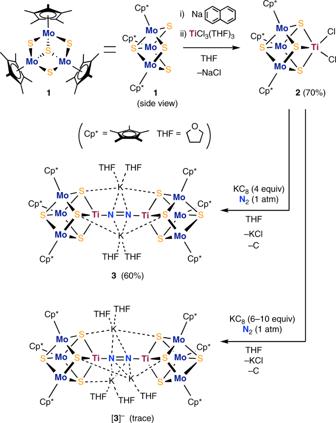Fig. 2 Reactions in this study. Synthesis of the cubic [Mo3S4Ti] cluster2, the N2-binding cluster3, and its 1e reduced form [3]–; Cp* = η5-pentamethylcyclopentadienyl; THF tetrahydrofuran 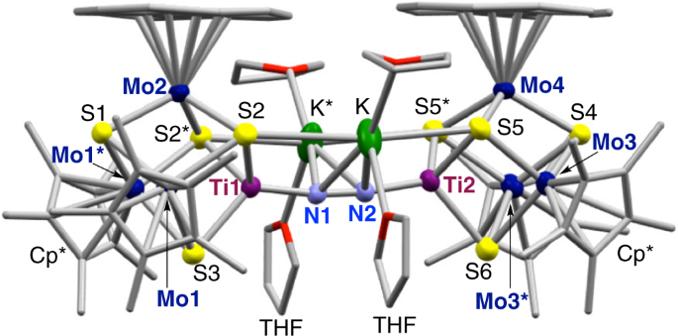Fig. 3 Molecular structure of the N2cluster3. For clarity, carbon and oxygen atoms are drawn as capped sticks, while other atoms are drawn with thermal ellipsoids set at 50% probability. Color legend: C, gray; Mo, dark blue; Ti, purple; S, yellow; O, red; N, light blue; K, green. Selected bond distances (Å): N1–N2 1.294(7), Mo1–Mo1* 2.6766(8), Mo1–Mo2 2.8853(6), Mo3–Mo3* 2.7392(8), Mo3–Mo4 2.8518(6), Mo1–Ti1 3.0315(10), Mo2–Ti1 3.0908(12), Mo3–Ti2 3.0301(10), Mo4–Ti2 3.0778(12), Ti1–N1 1.802(5), Ti2–N2 1.798(5), K–N1 2.797(3), K–N2 2.782(3) The molecular structure of 2 (Supplementary Figure 1 and Supplementary Table 3 ) reveals a nearly square-pyramidal geometry of titanium with an apical sulfur atom, where the Ti–S apical distance (2.2799(7) Å) is shorter than the Ti–S basal distances (2.3888(6) and 2.4272(6) Å). The Ti–Cl distances (2.3429(7) and 2.3812(7) Å) are close to those in a Ti(III) complex (average 2.353(4) Å) supported by three chlorides and a tridentate phosphine ligand [30] . The reduction of 2 with potassium graphite (KC 8 ) in THF under an atmosphere of N 2 resulted in the coordination and reduction of N 2 to form the brown cluster [K(THF) 2 ] 2 [Cp* 3 Mo 3 S 4 Ti] 2 (μ-N 2 ) ( 3 ) in 60% yield, in which an N 2 moiety bridges two [Mo 3 S 4 Ti] cubes via binding to the Ti atoms. Product(s) of analogous reactions under atmospheres of H 2 or Ar have not been characterized so far. Cluster 3 is diamagnetic, and the 15 N NMR spectrum of 15 N-labeled 3 exhibited a signal at –75.4 ppm relative to CH 3 NO 2 in THF- d 8 (Supplementary Figure 5 ). A single-crystal X-ray diffraction analysis of 3 established that N 2 is linearly aligned with the two Ti atoms to form a Ti–N=N–Ti moiety (Fig. 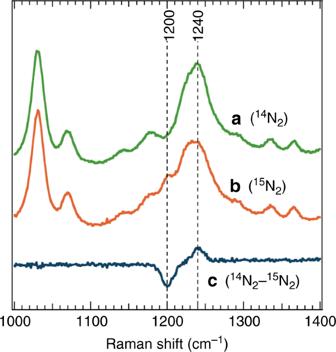Fig. 4 Spectroscopic characterization of the Ti-N=N-Ti moiety. Resonance-Raman spectra for3(a, green line) and15N-labeled3(b, orange line), as well as their difference spectrum (c, dark blue line) in THF at –30 °C 3 and Supplementary Figure 4 ). Its N–N distance (1.294(7) Å) is comparable to the longest bonds reported for Ti–N=N–Ti complexes [31] , [32] , [33] , suggesting a high degree of N 2 reduction. The N–N distance in 3 is slightly longer than that in H 3 CN=NCH 3 (1.25 Å) [34] , but shorter than that in H 2 N–NH 2 (1.46 Å) [25] , indicating a character between N=N double and N–N single bonds for the bridging N 2 in 3 . This notion was supported by resonance-Raman spectroscopy (Fig. 4 and Supplementary Figure 8 ), which showed a ν NN band of 3 at 1240 cm −1 based on the difference spectrum of 3 and 15 N-labeled 3 . This ν NN frequency falls between those of H 3 CN=NCH 3 (1575 cm −1 ) [35] and H 2 N–NH 2 (1111 cm −1 ) [36] . The observed shift (40 cm −1 ) between 3 (1240 cm −1 ) and 15 N-labeled 3 (1200 cm −1 ) is consistent with the calculated shift (42 cm −1 ) for the replacement of 14 N 2 by 15 N 2 assuming  a diatomic harmonic oscillator. Fig. 3 Molecular structure of the N 2 cluster 3 . For clarity, carbon and oxygen atoms are drawn as capped sticks, while other atoms are drawn with thermal ellipsoids set at 50% probability. Color legend: C, gray; Mo, dark blue; Ti, purple; S, yellow; O, red; N, light blue; K, green. Selected bond distances (Å): N1–N2 1.294(7), Mo1–Mo1* 2.6766(8), Mo1–Mo2 2.8853(6), Mo3–Mo3* 2.7392(8), Mo3–Mo4 2.8518(6), Mo1–Ti1 3.0315(10), Mo2–Ti1 3.0908(12), Mo3–Ti2 3.0301(10), Mo4–Ti2 3.0778(12), Ti1–N1 1.802(5), Ti2–N2 1.798(5), K–N1 2.797(3), K–N2 2.782(3) Full size image Fig. 4 Spectroscopic characterization of the Ti-N=N-Ti moiety. Resonance-Raman spectra for 3 ( a , green line) and 15 N-labeled 3 ( b , orange line), as well as their difference spectrum ( c , dark blue line) in THF at –30 °C Full size image Owing to the robust Cp*–Mo and Mo–S bonds in the present system, we speculate that the three Mo atoms remain intact during the activation of N 2 , leaving Ti as the reaction site in each cube. These robust bonds would also help to avoid the degradation of the cubic structure by aggregation or fragmentation. Conversion of the N 2 moiety into NH 3 and N 2 H 4 The high degree of reduction in 3 prompted us to attempt a stoichiometric conversion of the coordinated N 2 into NH 3 and N 2 H 4 . Upon treatment of 3 with protons from either H 2 O or HCl, the color changed from brown to green, and NH 3 , N 2 H 4 , and [ 1 ] + were detected. The resulting products NH 3 and N 2 H 4 were quantified by indophenol and azo-dye titration methods, respectively (Supplementary Tables 1 and 2 ) [37] , [38] . As summarized in Table 1 (entries 1 and 4), small to moderate amounts of NH 3 (0.12(3)–0.29(5) equiv) and N 2 H 4 (0.12(10)–0.60(3) equiv) were detected by protonation of 3 with an excess H 2 O or HCl. While the length of the N–N bond in 3 indicates that a reduction has occurred, additional electrons are required for the cleavage of the N–N bond to form NH 3 . Therefore 3 was treated with KC 8 and H 2 O or HCl. In the presence of 6 equiv of KC 8 , the average amount of NH 3 generated by protonation with H 2 O increased from 0.12(3) to 0.47(27) equiv (entry 5), while the fluctuations observed allow only a cautious comparison. The NH 3 yields in entries 4 and 5 (HCl) are comparable and within error. The yields of N 2 H 4 in entries 2 (0.56(10) equiv from H 2 O) and 5 (0.19(6) equiv from HCl) remained comparable to those of reactions in the absence of KC 8 . The formation of N 2 H 4 from the Ti–N=N–Ti moiety is reasonable, as this N–N bond exhibits an N=N double and N–N single bond character. In the presence of 0–6 equiv of KC 8 , subsequent protonation by H 2 O provided approximately three times the amount of N 2 H 4 than the reactions with HCl. Such acid-dependent selectivity may arise from the affinities of the conjugate bases (OH – or Cl – ) toward metals, where the high oxophilicity of the Ti and K atoms can facilitate the coordination of H 2 O onto these atoms, which could lead to an efficient protonation of the neighboring Ti–N=N–Ti moiety. Table 1 Protonation of 3 in the presence/absence of KC 8 a Full size table Even in the presence of a slight excess (6 equiv) of KC 8 , conversion of the N 2 moiety of 3 into NH 3 was not complete and notable amounts of N 2 H 4 were detected (entries 2 and 5). These results indicate that some of the added KC 8 remains unreacted with the N 2 cluster and is subsequently quenched directly by H 2 O or HCl. However, the formation of N 2 H 4 was suppressed when a large excess of KC 8 was added prior to protonation (entries 3 and 6). While the protonation with HCl did not increase the amount of NH 3 (entry 6), the maximum yield of NH 3 (1.20(19) equiv) was achieved when 100 equiv KC 8 were added prior to the protonation with H 2 O (entry 3). When conditions identical to those of entry 3 were applied for the 15 N-enriched 3 under an atmosphere of 14 N 2 , the 1 H NMR spectrum of the resulting ammonium salt indicated the exclusive formation of 15 NH 3 , which originates from the Ti– 15 N= 15 N–Ti moiety (Supplementary Figure 15 ). After addition of an excess of protons to 3 , the Ti atom probably dissociates from the [Mo 3 S 4 Ti] cube, which is supported by the appearance of an intense signal of [ 1 ] + in the electro-spray ionization mass (ESI-MS) spectrum of the resulting mixture (Supplementary Figure 16 ) and the color change of the mixture from dark brown to green. Thus, at this stage, the possibility of N 2 functionalization after dissociation of the Ti atom cannot be ruled out unequivocally. It has been reported that metal–sulfur clusters exhibit stability across various oxidation states, which allows the storage and transportation of electrons [39] , [40] . It is therefore worthy of notice that the 1e-reduced cluster [ 3 ] – was obtained in trace amounts from the reaction of 2 with 6–10 equiv of KC 8 under an atmosphere of N 2 (Fig. 2 , bottom). The characterization of [ 3 ] – was carried out only by 1 H NMR and crystallographic analysis due to the trace amounts available. Cluster [ 3 ] – is paramagnetic and its 1 H NMR spectrum in THF- d 8 exhibited a broad Cp* signal at 5.84 ppm (Supplementary Figure 10 ). The molecular structure of [ 3 ] – (Supplementary Figure 9 ) revealed an interaction of three potassium ions with the bridging N 2 moiety, where the N–N distance (1.293(5) Å) is comparable to that in 3 (1.294(7) Å). A structural comparison between the [Mo 3 S 4 Ti] cubes of 3 and [ 3 ] – reveals the elongation of distances in [ 3 ] – . In detail, a relatively large contribution of the metal atoms for the storage of the additional electron is indicated by the larger differences in the average distances of Mo–Ti (3.0487(12) Å for 3 and 3.0242(8) Å for [ 3 ] – ) and Mo–Mo (2.8150(8) Å for 3 and 2.8668(6) Å for [ 3 ] – ), rather than the average metal–sulfur distances, i.e. Mo–S (2.3952(16) Å for 3 and 2.3966(11) Å for [ 3 ] – ), and Ti–S (2.328(2) Å for 3 and 2.3297(13) Å for [ 3 ] – ). The detailed reaction pathways for the formation of NH 3 and N 2 H 4 from 3 or [ 3 ] – remain unclear at this point, as the dissociation of the Ti atom from the [Mo 3 S 4 Ti] cube renders the identification of possible cluster intermediates difficult. In summary, we successfully achieved the activation of N 2 and its conversion into sub-stoichiometric mixtures of NH 3 and N 2 H 4 on synthetic Mo–Ti–S cubes by selectively generating the Ti-based reaction sites. This work thus represents a step towards the assembly of structural and functional models for the FeMo-cofactor. General procedure All reactions and manipulations were carried out under an atmosphere of nitrogen using standard Schlenk line or glove box techniques. Solvents for reactions were purified by passing over columns of activated alumina and a supported copper catalyst. TiCl 3 (THF) 3 [41] , [Cp* 3 Mo 3 S 4 ][PF 6 ] ([ 1 ] + ) [42] , and KC 8 [43] were prepared according to literature procedures. All other reagents were purchased from common commercial sources and used without further purification. General considerations on the measurements and experiments as well as some experimental details are described in the Supplementary Methods . Modified synthesis of Cp* 3 Mo 3 S 4 (1) Compound 1 was originally synthesized from the reaction of Cp*Mo(S t Bu) 3 ( t Bu = tert -butyl) with Na/Hg [24] , but this reaction is not ideally suitable for a gram-scale synthesis. Instead, cluster 1 was synthesized on a multi-gram scale through the reduction of [ 1 ] + . For that purpose, KC 8 (1.36 g, 10.06 mmol) was added in portions to a THF (150 mL) suspension of [ 1 ] + (9.78 g, 10.12 mmol) at room temperature. After stirring this mixture overnight, the solvent was removed under reduced pressure. The residue was extracted four times with toluene (350 mL). The extract was stored at –30 °C to precipitate green blocks of 1 . The mother liquor was concentrated to ca. 1/5 of the original volume and stored at –30 °C to obtain a second crop. The total amount of green crystals of 1 was 6.17 g (7.51 mmol, 83%). This product was characterized by comparison with 1 H NMR data in the literature [24] . 1 H NMR (C 6 D 6 ): δ 8.56 ( w 1/2 = 14 Hz, Cp*). Synthesis of Cp* 3 Mo 3 S 4 TiCl 2 (2) A THF (20 mL) solution of 1 (1.00 g, 1.22 mmol) was cooled to –100 °C, and a THF solution of sodium naphthalenide (19.5 mM, 62 mL, 1.21 mmol) was added. The reaction mixture was gradually warmed to room temperature to give a dark green solution. The mixture was again cooled to –100 °C, and TiCl 3 (THF) 3 (451 mg, 1.22 mmol) was added. The reaction mixture was warmed to room temperature and stirred for 5 days, affording a dark brown suspension. After concentration to ca. 5 mL under reduced pressure, the mixture was cooled to –30 °C, which caused the precipitation of a dark brown powder. The supernatant was removed and the dark brown powder was washed with hexane (20 mL × 2). The brown powder was dissolved into CH 2 Cl 2 (15 + 3 mL), and hexane (100 mL) was layered on top of this solution. The subsequent slow diffusion led to the formation of brown plates of Cp* 3 Mo 3 S 4 TiCl 2 · CH 2 Cl 2 ( 2· CH 2 Cl 2 ). These  brown crystals were washed with hexane (15 mL × 2), and then dissolved in THF (15 mL). After stirring overnight, THF and CH 2 Cl 2 were removed under reduced pressure to give a brown powder of 2 (801 mg, 0.854 mmol, 70%). 1 H NMR (CD 2 Cl 2 ): δ 9.23 ( w 1/2 = 8 Hz, Cp*); solution magnetic moment (CD 2 Cl 2 , 297 K): μ eff = 1.3 μ B ; Cyclic voltammogram (2 mM in CH 2 Cl 2 , potential vs. (C 5 H 5 ) 2 Fe/[(C 5 H 5 ) 2 Fe] + ): E 1/2 = –0.28, –1.34 V; UV/Vis (CH 2 Cl 2 ): λ max 415 nm (sh, 1200 cm −1 M −1 ), 753 nm (660 cm −1 M −1 ); analysis (calcd., found for C 30 H 45 Cl 2 Mo 3 S 4 Ti): C (38.31, 38.77), H (4.82, 4.70), S (13.64, 13.24). Synthesis of [K(THF) 2 ] 2 [Cp* 3 Mo 3 S 4 Ti] 2 (μ-N 2 ) (3) Cluster 2 (200 mg, 0.213 mmol) and KC 8 (116 mg, 0.858 mmol) were charged into one side of an H-shaped glass vessel (Supplementary Fig. 3 ). The other arm of the vessel was charged with THF (10 mL), which was vacuum-transferred to the solid mixture at 78 K. The vessel was filled with N 2 (1 atm) and then sealed. The mixture was slowly warmed using a methanol/liquid N 2 slurry. Stirring of the mixture with a magnetic stirring bar was initiated, once part of frozen THF had melted. The mixture was gradually warmed to room temperature, giving a dark red-brown suspension. Stirring was continued overnight, before the solvent was removed under reduced pressure and the residue was extracted with THF (50 mL). The solution was filtered, concentrated to ca. 3 mL, and stored at –30 °C. Cluster 3 (136 mg, 0.064 mmol, 60%) was obtained as dark-brown crystalline blocks, which were washed with pentane. 1 H NMR (THF- d 8 ): δ 1.70 (Cp*); 13 C{ 1 H} NMR (THF- d 8 ): δ 13.6 (C 5 Me 5 ), 96.3 ( C 5 Me 5 ); UV/Vis (THF): λ max 356 nm (35800 cm −1 M −1 ), 500 nm (15,800 cm −1 M −1 ); Resonance-Raman spectrum (0.07 mM in THF, λ ex 355 nm, –30 °C): 1240 cm -1 ( ν NN ); analysis (calcd., found for C 76 H 122 K 2 Mo 6 N 2 O 4 S 8 Ti 2 ): C (42.78, 42.36), H (5.76, 5.80), N (1.31, 1.37), S (12.02, 12.27). Synthesis of 15 N 2 -labeled 3 This cluster was synthesized in a manner similar to that of 3 , using cluster 2 (173 mg, 0.184 mmol), KC 8 (100 mg, 0.740 mmol), and 15 N 2 (1 atm). Crystals of 15 N 2 -labeled 3 were obtained in 60% yield (117 mg, 0.055 mmol). 15 N{ 1 H} NMR (THF- d 8 , referenced to external CH 3 NO 2 ): δ –75.4; Resonance-Raman spectrum (THF, –30 °C): 1200 cm −1 ( ν NN ). Data availability The X-ray crystallographic coordinates for structures reported in this study have been deposited at the Cambridge Crystallographic Data Centre (CCDC), under deposition numbers 1577330–1577332. These data can be obtained free of charge from The Cambridge Crystallographic Data Centre via www.ccdc.cam.ac.uk/data_request/cif . All other data are available from the authors upon request.